Mutations in thePQBP1gene prevent its interaction with the spliceosomal protein U5–15kD A loss-of-function of polyglutamine tract-binding protein 1 (PQBP1) induced by frameshift mutations is believed to cause X-linked mental retardation. However, the mechanism by which structural changes in PQBP1 lead to mental retardation is unknown. Here we present the crystal structure of a C-terminal fragment of PQBP1 in complex with the spliceosomal protein U5–15kD. The U5–15kD hydrophobic groove recognizes a YxxPxxVL motif in PQBP1, and mutations within this motif cause a loss-of-function phenotype of PQBP1 in vitro . The YxxPxxVL motif is absent in all PQBP1 frameshift mutants seen in cases of mental retardation. These results suggest a mechanism by which the loss of the YxxPxxVL motif could lead to the functional defects seen in this type of mental retardation. The splicing of precursor messenger RNA (pre-mRNA) is a process that removes non-coding introns and splices together exons in newly transcribed pre-mRNA. The pre-mRNA splicing is catalysed by the spliceosome, a multimegadalton ribonucleoprotein complex comprising RNA–protein complexes termed uridine-rich small nuclear ribonucleoprotein particles (U snRNPs), namely, the U1, U2, U4, U5 and U6 snRNPs [1] , [2] , [3] . Spliceosome assembly is known to proceed in a dynamic manner: the snRNP and non-snRNP splicing factors dynamically associate and dissociate, accompanied by structural rearrangements. During the assembly process, there are five distinct stages that are commonly designated as the E, A, B, B* and C complexes. These complexes comprise one or more U snRNPs in complex with the pre-mRNA [1] , [2] , [3] . The prespliceosomal A complex contains U1 and U2 snRNPs and proteins involved in early recognition of the splice sites. The A complex recruits the preformed U4/U6.U5 tri-snRNP to form the precatalytic B complex. The B complex subsequently undergoes major rearrangements, including destabilization or loss of the U1 and U4 snRNPs, leading to catalytic activation and formation of the so-called activated spliceosome (B* complex). The B* spliceosome catalyses the first step of pre-mRNA splicing. The second step of the catalytic reaction takes place in the C complex that is generated by reorganization of the B* complex. After the second step, mRNA is released and the postspliceosomal complex, which contains the excised intron and the U2, U5 and U6 snRNPs, is disassembled [1] , [2] , [3] . The polyglutamine tract-binding protein 1 (PQBP1), also known as Npw38, is one of the pre-mRNA splicing factors involved in the precatalytic B complex [4] , [5] . PQBP1 interacts with many proteins, including the U5 snRNP-specific 15kD protein (U5–15kD) [6] , [7] , [8] and WBP11/NpwBP/SIPP1 (ref. 9 ). U5–15kD specifically interacts with the C-terminal domain of PQBP1 (refs 6 , 7 ), while WBP11 interacts with the WW domain of PQBP1 (ref. 9 ). However, the function of PQBP1 in pre-mRNA splicing remains unclear. A number of studies have indicated that the PQBP1 gene is causative for X-linked mental retardation (XLMR) disorders, such as the Renpenning, Sutherland-Haan, Hamel, Porteous and Golabi-Ito-Hall syndromes [10] , [11] , [12] , [13] , [14] , [15] , [16] , [17] , [18] . Patients with these diseases frequently share similar symptoms, such as intellectual disability, microcephaly and short stature. So far, 11 mutations associated with XLMR have been identified in the PQBP1 gene. One is a missense mutation in which the conserved Tyr65 in the WW domain is changed to Cys [14] . And another is a deletion of 21 base pairs that results in the loss of seven amino acids in the polar amino-acid-rich domain [10] . The most common type are frameshift mutations causing a premature termination codon. Such frameshift mutations result in partial or total loss of the C-terminal domain that is functionally important for the interaction between PQBP1 and the spliceosomal U5–15kD [10] , [11] , [12] , [13] , [15] , [16] , [17] , [18] . Based on these findings, the loss of function of PQBP1 in the pre-mRNA splicing is believed to cause XLMR [12] , [19] , [20] , [21] , [22] . However, the structural mechanism by which the PQBP1 loss-of-function causes pre-mRNA splicing defects is unknown. Here we present the crystal structure of a C-terminal fragment of PQBP1 in complex with the spliceosomal U5–15kD. In addition, we reveal the structure of the heterotrimer formed by the PQBP1 C-terminal fragment, U5–15kD, and the U5 snRNP-specific 52K protein (U5–52K). From the crystal structures of the complexes and the interaction analysis, we find that the YxxPxxVL motif in PQBP1 is essential for maintaining the complex involving PQBP1. We also find that the frameshift mutations cause the loss of a YxxPxxVL motif in PQBP1. These results suggest a mechanism by which the loss of the YxxPxxVL motif could lead to the functional defects seen in this type of mental retardation. The binary complex of PQBP1 and U5–15kD PQBP1 is composed of a small folded WW domain and long unstructured regions containing the polar amino-acid-rich domain and the C-terminal domain ( Fig. 1 ) [23] , [24] . To crystallize the complex of PQBP1 and U5–15kD, we used a C-terminal 43-residue fragment of PQBP1 (PQBP1-CT43). We have previously shown that free PQBP1-CT43 is intrinsically disordered in solution [24] . The binary complex of PQBP1-CT43 and U5–15kD was obtained by mixing the proteins at a 1:5 molar ratio (U5–15kD to PQBP1-CT43). The crystals belong to space group P2 and contain four heterodimeric complexes in the asymmetric unit. 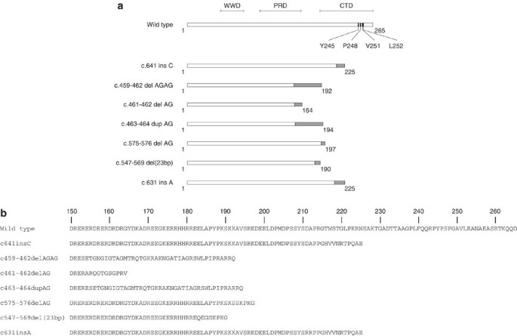Figure 1: Comparison of the amino-acid sequences of wild-type PQBP1 and the frameshift mutants causing mental retardation. These frameshift mutations generate premature termination codons, causing the truncation of PQBP1. (a) The grey bars represent the positions where amino acids are changed by the frameshift mutations. The positions of Tyr245, Pro248, Val251 and Leu252 are shown in wild-type PQBP1. The positions of the functional domain of PQBP1 are indicated above the figure. WWD, WW domain; PRD, polar amino-acid-rich domain; and CTD, C-terminal domain. (b) Partial amino-acid sequences of wild-type PQBP1 and the frameshift mutants causing mental retardation. The crystal structure of the binary complex was refined to a resolution of 2.1 Å with an R work / R free value of 19/25% ( Table 1 ). The refined model of the PQBP1-CT43 in the complex consists of the residues 238–260: it lacks the 15 N-terminal residues (residues 223–237; KRNEAKTGADTTAAG) and the 5 C-terminal residues (residues 261–265; TKQQD) owing to conformational flexibility ( Fig. 2a ). PQBP1-CT43 in the complex adopts an L-shaped structure with an extended conformation (residues 238–247) followed by an α-helix conformation (residues 248–259). The α-helix starts at Pro248, which generates the bend of the L-shaped structure. The complex is mainly stabilized by hydrophobic contacts that include Tyr245, Pro248, Val251 and Leu252 of PQBP1 interacting with Val14, Ile18, Phe69, Met72, Tyr73, Met82 and Phe84 in the hydrophobic groove of U5–15kD ( Fig. 2b,d ). In addition, two hydrogen bonds stabilize the complex: the hydrogen bond between Tyr245 (PQBP1) and Glu74 (U5–15kD) and that between Asn255 (PQBP1) and Asp68 (U5–15kD) ( Fig. 2a,c ). The F O − F C difference electron density map for PQBP1-CT43 before its inclusion in refinement reveals the electron density for Tyr245, Pro248, Val251, Leu252 and Asn255 of PQBP1-CT43 ( Supplementary Fig. 1 ). The total surface area buried upon complex formation is 1,354.2 Å 2 . Figure 1: Comparison of the amino-acid sequences of wild-type PQBP1 and the frameshift mutants causing mental retardation. These frameshift mutations generate premature termination codons, causing the truncation of PQBP1. ( a ) The grey bars represent the positions where amino acids are changed by the frameshift mutations. The positions of Tyr245, Pro248, Val251 and Leu252 are shown in wild-type PQBP1. The positions of the functional domain of PQBP1 are indicated above the figure. WWD, WW domain; PRD, polar amino-acid-rich domain; and CTD, C-terminal domain. ( b ) Partial amino-acid sequences of wild-type PQBP1 and the frameshift mutants causing mental retardation. Full size image Table 1 Data collection and refinement statistics. 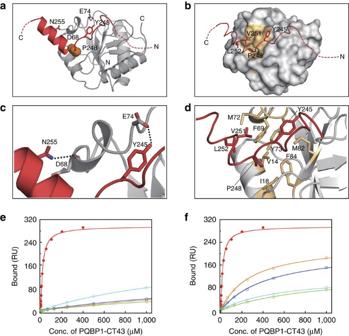Figure 2: Characterization of the binary complex of PQBP1-CT43 and U5–15kD. (a–d) Structure of the binary complex of PQBP1-CT43 (red) and U5–15kD (grey). The disordered regions are depicted with dashed lines. (a,c) Hydrogen bonds are indicated by dotted lines. Asn255 and Tyr245 of PQBP1-CT43 and Asp68 and Glu74 of U5–15kD are shown in stick mode. The side chain of Pro248 is shown as a sphere (orange). (b,d) The side chains of Tyr245, Pro248, Val251 and Leu252 of PQBP1-CT43 are shown in stick mode. The orange-colored surface and sticks indicate the positions of Val14, Ile18, Phe69, Met72, Tyr73, Met82 and Phe84 in the hydrophobic groove of U5–15kD. (e,f) Equilibrium binding curves of PQBP1-CT43 to the biotinylated U5–15kD. The binding response at equilibrium was plotted against the concentration (Conc.) of PQBP1-CT43. The data were fitted to a 1:1 Langmuir binding model (solid lines). The experiments were repeated at least three times and the average of the dissociation constants±s.d. is presented inTables 2and3. (e) Equilibrium binding curves of the Asp-mutants to U5–15kD. Red, wild-type PQBP1-CT43; cyan, Y245D; orange, P248D; blue, V251D; and green, L252D. (f) Equilibrium binding curves of the Ala-mutants to U5–15kD. Red, wild-type PQBP1-CT43; cyan, Y245A; orange, P248A; blue, V251A; and green, L252A. Full size table Figure 2: Characterization of the binary complex of PQBP1-CT43 and U5–15kD. ( a – d ) Structure of the binary complex of PQBP1-CT43 (red) and U5–15kD (grey). The disordered regions are depicted with dashed lines. ( a , c ) Hydrogen bonds are indicated by dotted lines. Asn255 and Tyr245 of PQBP1-CT43 and Asp68 and Glu74 of U5–15kD are shown in stick mode. The side chain of Pro248 is shown as a sphere (orange). ( b , d ) The side chains of Tyr245, Pro248, Val251 and Leu252 of PQBP1-CT43 are shown in stick mode. The orange-colored surface and sticks indicate the positions of Val14, Ile18, Phe69, Met72, Tyr73, Met82 and Phe84 in the hydrophobic groove of U5–15kD. ( e , f ) Equilibrium binding curves of PQBP1-CT43 to the biotinylated U5–15kD. The binding response at equilibrium was plotted against the concentration (Conc.) of PQBP1-CT43. The data were fitted to a 1:1 Langmuir binding model (solid lines). The experiments were repeated at least three times and the average of the dissociation constants±s.d. is presented in Tables 2 and 3 . ( e ) Equilibrium binding curves of the Asp-mutants to U5–15kD. Red, wild-type PQBP1-CT43; cyan, Y245D; orange, P248D; blue, V251D; and green, L252D. ( f ) Equilibrium binding curves of the Ala-mutants to U5–15kD. Red, wild-type PQBP1-CT43; cyan, Y245A; orange, P248A; blue, V251A; and green, L252A. Full size image We also solved the structure of a fusion protein of U5–15kD(4–137) and PQBP1-CT43 ( Supplementary Fig. 2 ). PQBP1-CT43 was fused to the C terminus of U5–15kD(4–137) without an additional linker sequence, as the N-terminal 15 residues of PQBP1-CT43 are disordered in the binary complex ( Fig. 2a ). The crystal structure of the fusion protein was refined to a resolution of 2.5 Å with an R work / R free value of 19/24% ( Table 1 ). The refined model of the fusion protein is missing the residues 223–243 and 260–265 of PQBP1, presumably owing to conformational flexibility. The linking of PQBP1-CT43 with U5–15kD(4–137) did not affect those structures of Tyr245, Pro248, Val251 and Leu252 of PQBP1 that interact with the hydrophobic groove of U5–15kD ( Supplementary Fig. 2 ). To evaluate the affinity of PQBP1-CT43 and U5–15kD, we performed surface plasmon resonance (SPR) measurements. PQBP1-CT43 at various concentrations was injected over sensor surfaces on which the biotinylated U5–15kD had been immobilized ( Fig. 2e,f ). The binding curve was analysed by assuming a 1:1 Langmuir binding model. The equilibrium dissociation constant ( K D ) between PQBP1-CT43 and U5–15kD was determined to be 19.7±3.4 μM. The K D value was confirmed by fluorescence measurements (24.4±3.4 μM; Supplementary Fig. 3b ). We also used SPR to determine the K D value between full-length PQBP1 and U5–15kD, which was 26.1±2.8 μM. In addition, fluorescence anisotropy measurements showed that full-length PQBP1 binds to U5–15kD with a K D value of 25.7±3.9 μM ( Supplementary Fig. 3a ). These results indicate that the C-terminal 43-residue fragment is sufficient for the interaction. PQBP1 binds to U5–15kD via its YxxPxxVL motif To validate the interactions between PQBP1-CT43 and U5–15kD, we used site-directed mutagenesis of PQBP1-CT43 ( Fig. 2e,f ). The mutagenesis was designed to change the residues that are in contact with U5–15kD. Table 2 summarizes the K D values of the mutants in which the residues are replaced by Asp. The Asp mutation was used to disrupt the hydrophobic contacts between PQBP1 and U5–15kD, as Asp is a small amino acid and is very polar. Mutagenesis of the PQBP1 interface residues Tyr245, Pro248, Val251 and Leu252 to Asp clearly showed the importance of the hydrophobic contacts for the interaction between PQBP1-CT43 and U5–15kD ( Fig. 2e ; Table 2 ). In addition, we performed site-directed Ala mutagenesis and showed the importance of Tyr245, Pro248, Val251 and Leu252 for the interaction ( Fig. 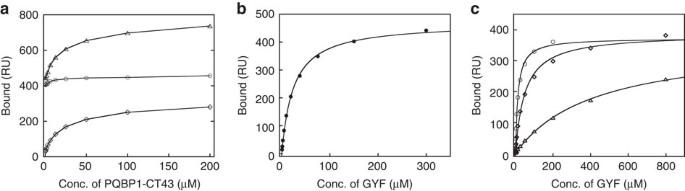Figure 3: SPR analysis of the interactions between PQBP1, U5–15kD and the GYF domain of U5–52K. (a) Competitive binding of PQBP1-CT43 and the GYF domain of U5–52K to the biotinylated U5–15kD. The GYF domain (120 μM) was preincubated with varying concentrations (Conc.) of PQBP1-CT43 (0.4−200 μM) for at least 30 min, and the mixture was injected over the immobilized U5–15kD. The binding response at equilibrium was plotted against the concentration of PQBP1-CT43. The responses in the absence and presence of the GYF domain are indicated by diamonds and triangles, respectively. The differences between the responses in the presence and absence of the GYF domain are indicated by circles. (b,c) Equilibrium binding curves of the GYF domain of U5–52K to the biotinylated U5–15kD and U5–15kD-PQBP1-CT43. The binding response at equilibrium was plotted against the concentration of the GYF domain. The data were fitted to a 1:1 Langmuir binding model (solid lines). The experiments were repeated at least three times and the average of the dissociation constants±s.d. is presented. (b) Equilibrium binding curves of the GYF domain to U5–15kD. TheKDbetween the GYF domain and U–15kD is 23.1±1.3 μM. (c) Equilibrium binding curves of the GYF domain to U5–15kD-PQBP1-CT43. Circles, wild-type GYF domain; triangles, Y330A-GYF; and diamonds, L339A-GYF. TheKDbetween the GYF domain and U5-15kD-PQBP1-CT43 is 12.9±0.2 μM. TheKDvalues of Y330A-GYF and L339A-GYF are 421±28.3 and 49.8±2.8 μM, respectively. 2f ; Table 3 ). From these results, we defined the YxxPxxVL motif in PQBP1 as a U5–15kD-binding motif. Intriguingly, the YxxPxxVL motif is lost in all the PQBP1 frameshift mutants responsible for mental retardation ( Fig. 1 ). This means that the frameshift mutations in the PQBP1 gene cause the loss of the YxxPxxVL motif that is essential for the U5–15kD binding. The Y245A and L252A mutations resulted in a large reduction in the affinity between PQBP1-CT43 and U5–15kD. The buried surface areas of Tyr245 and Leu252 are 185.0 and 87.5 Å 2 , respectively, which correspond to 27 and 13% of the buried surface area of PQBP1-CT43 upon binding to U5–15kD. Table 2 The equilibrium dissociation constants between the Asp-mutants of PQBP1-CT43 and U5–15kD (pH 8.5 and 25 °C). Full size table Table 3 The equilibrium dissociation constants between the Ala-mutants of PQBP1-CT43 and U5–15kD (pH 8.5 and 25 °C). Full size table We also determined the K D values of the PQBP1 mutants in which the neighbouring residues were replaced by Asp. The mutation of Arg253 and Asn255 to Asp significantly reduced the affinity between PQBP1-CT43 and U5–15kD ( Table 2 ). However, the mutation of Arg253 and Asn255 to Ala had only slight effects on the affinity, indicating that these residues made only a minor contribution to the interaction ( Table 3 ). The ternary complex of PQBP1, U5–15kD and U5–52K It is known that U5–15kD interacts with U5–52K as well as PQBP1 (ref. 25 ). This interaction is mediated by the Glu111-Ser132 of U5–15kD and a C-terminal GYF domain (residues 280–341) of U5–52K (ref. 26 ). Although PQBP1 and U5–52K bind to different surfaces of U5–15kD [24] , it is not clear whether PQBP1 and U5–52K interfere with each other when binding to U5–15kD. Hence, we next investigated whether PQBP1-CT43 could compete with the GYF domain of U5–52K to bind to U5–15kD. We performed a competitive binding experiment in which a mixture of PQBP1-CT43 and the GYF domain was injected over sensor surfaces on which the biotinylated U5–15kD had been immobilized ( Fig. 3a ). The concentration of PQBP1-CT43 was set to 0.4−200 μM, whereas the concentration of the GYF domain was constant (120 μM). The difference between the responses in the presence and absence of the GYF domain was almost constant (430 response units), indicating that PQBP1-CT43 does not compete with the GYF domain. Figure 3: SPR analysis of the interactions between PQBP1, U5–15kD and the GYF domain of U5–52K. ( a ) Competitive binding of PQBP1-CT43 and the GYF domain of U5–52K to the biotinylated U5–15kD. The GYF domain (120 μM) was preincubated with varying concentrations (Conc.) of PQBP1-CT43 (0.4−200 μM) for at least 30 min, and the mixture was injected over the immobilized U5–15kD. The binding response at equilibrium was plotted against the concentration of PQBP1-CT43. The responses in the absence and presence of the GYF domain are indicated by diamonds and triangles, respectively. The differences between the responses in the presence and absence of the GYF domain are indicated by circles. ( b , c ) Equilibrium binding curves of the GYF domain of U5–52K to the biotinylated U5–15kD and U5–15kD-PQBP1-CT43. The binding response at equilibrium was plotted against the concentration of the GYF domain. The data were fitted to a 1:1 Langmuir binding model (solid lines). The experiments were repeated at least three times and the average of the dissociation constants±s.d. is presented. ( b ) Equilibrium binding curves of the GYF domain to U5–15kD. The K D between the GYF domain and U–15kD is 23.1±1.3 μM. ( c ) Equilibrium binding curves of the GYF domain to U5–15kD-PQBP1-CT43. Circles, wild-type GYF domain; triangles, Y330A-GYF; and diamonds, L339A-GYF. The K D between the GYF domain and U5-15kD-PQBP1-CT43 is 12.9±0.2 μM. The K D values of Y330A-GYF and L339A-GYF are 421±28.3 and 49.8±2.8 μM, respectively. Full size image In addition, we solved the structure of a heterotrimer of PQBP1, U5–15kD, and the GYF domain of U5–52K. In order to crystallize the heterotrimer, we first used the fusion protein of U5–15kD(4–137) and PQBP1-CT43, which was complexed with the GYF domain of U5–52K. As described above, the linking of PQBP1-CT43 with U5–15kD(4–137) did not affect the structure of the YxxPxxVL motif in PQBP1 ( Supplementary Fig. 2 ). Although the complex formed with the fusion protein (U5–15kD-PQBP1-CT43) and the GYF domain was crystallized, the diffraction quality of the crystal was greatly improved by shortening the disordered region of PQBP1. Therefore, a C-terminal 37-residue fragment of PQBP1 (PQBP1-CT37) was fused to the C terminus of U5–15kD without an additional linker sequence, and the fusion protein was complexed with the GYF domain of U5–52 K at a 1:1 molar ratio ( Fig. 4a ). The crystals belong to space group I2 and contain two heterotrimeric complexes in the asymmetric unit. The crystal structure of the ternary complex was refined to a resolution of 2.5 Å with an R work / R free value of 24/28% ( Table 1 ). The overall conformations of the PQBP1 C-terminal fragment and U5–15kD did not change in the presence of the GYF domain, which is consistent with the competitive binding experiment. The refined model of PQBP1-CT37 lacks the N-terminal nine residues (residues 229–237; TGADTTAAG) and the C-terminal five residues (TKQQD) owing to conformational flexibility. The GYF domain and the U5–15kD are bound mainly by polar interactions ( Fig. 4b ). Hydrophobic contact makes only a minor contribution to the interaction between U5–15kD and the GYF domain [26] . The total buried surface area upon binding of the GYF domain to U5–15kD is 1,228.6 Å 2 , which is similar to the total buried surface area upon binding of PQBP1-CT37 to U5–15kD (1,349.6 Å 2 ). The total buried surface areas are compatible with the binding affinities of U5–15kD for the GYF domain and for PQBP1: the K D value between U5–15kD and the GYF domain was determined to be 23.1±1.3 μM ( Fig. 3b ), which was comparable to the K D value for the interaction between U5–15kD and PQBP1-CT43 (19.7±3.4 μM). 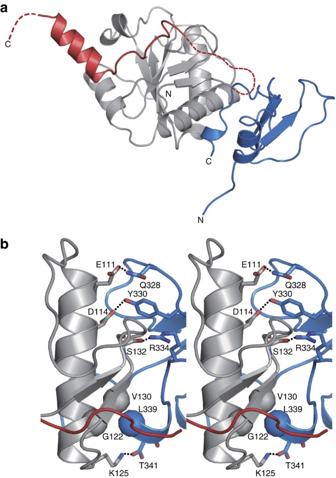Figure 4: Structure of the ternary complex of PQBP1-CT37 (red), U5–15kD (grey) and the GYF domain of U5–52K (blue). (a) The disordered regions are depicted with dashed lines. PQBP1-CT37 is fused to the C terminus of U5–15kD. The fusion protein is complexed with the GYF domain at a 1:1 molar ratio. (b) Interface between U5–15kD and the GYF domain showing hydrogen bonds (dotted lines) and hydrophobic contacts (spheres). Glu111, Asp114, Ser132 and Lys125 of U5–15kD and Gln328, Tyr330, Arg334 and Thr341 of U5–52K are shown in stick mode. The α-carbons of Leu339 (U5–52K), Val130 (U5–15kD) and Gly122 (U5–15kD) are shown as spheres. A hydrogen bond between the carboxylate oxygen of the C-terminal Thr341 (U5–52K) and the side chain of Lys125 (U5–15kD) is also indicated by a dotted line. Figure 4: Structure of the ternary complex of PQBP1-CT37 (red), U5–15kD (grey) and the GYF domain of U5–52K (blue). ( a ) The disordered regions are depicted with dashed lines. PQBP1-CT37 is fused to the C terminus of U5–15kD. The fusion protein is complexed with the GYF domain at a 1:1 molar ratio. ( b ) Interface between U5–15kD and the GYF domain showing hydrogen bonds (dotted lines) and hydrophobic contacts (spheres). Glu111, Asp114, Ser132 and Lys125 of U5–15kD and Gln328, Tyr330, Arg334 and Thr341 of U5–52K are shown in stick mode. The α-carbons of Leu339 (U5–52K), Val130 (U5–15kD) and Gly122 (U5–15kD) are shown as spheres. A hydrogen bond between the carboxylate oxygen of the C-terminal Thr341 (U5–52K) and the side chain of Lys125 (U5–15kD) is also indicated by a dotted line. Full size image We evaluated the affinity between the fusion protein (U5–15kD-PQBP1-CT43) and the GYF domain using SPR ( Fig. 3c ). The GYF domain was injected over sensor surfaces on which the biotinylated U5–15kD-PQBP1-CT43 had been immobilized. We determined the K D value between the GYF domain and U5–15kD-PQBP1-CT43, which was 12.9±0.2 μM ( Fig. 3c ). Therefore, PQBP1 does not inhibit the binding of U5–52K to U5–15kD, which is consistent with the competitive binding experiment. In addition, single mutations (Y330A and L339A in U5–52K) reduced the affinity between U5–15kD-PQBP1-CT43 and the GYF domain ( Fig. 3c ). This observation is consistent with the heterotrimeric structure: Tyr330 (U5–52K) forms a hydrogen bond with Asp114 (U5–15kD) and Leu339 (U5–52K) forms hydrophobic contacts with Val130 (U5–15kD) and Gly122 (U5–15kD) ( Fig. 4b ). Alternative splicing is a process by which exons are joined in different ways during pre-mRNA splicing [27] . More than 70% of human pre-mRNAs undergo alternative splicing to produce various protein isoforms [2] . It is becoming evident that aberrant alternative splicing leads to various human diseases, particularly neurological diseases [28] , [29] , [30] . PQBP1 is dominantly expressed in the central nervous system in embryos and in newborn mice [20] , and PQBP1 knockdown results in impairment of anxiety-related cognition and memory [19] . A recent study by Wang et al. [22] has shown that PQBP1 knockdown in primary mouse neurons results in aberrant alternative splicing of pre-mRNAs that are important for neuron projection development, although the precise mechanism by which this occurs remains to be explored. In addition, Ikeuchi et al. [31] have identified a function for PQBP1 in the morphogenesis of the primary cilium in postmitotic neurons. In their study, knockdown of PQBP1 profoundly impaired the formation of the primary cilium in hippocampal neurons and the mouse cerebral cortex in vivo [31] . These results suggest that the loss of function of PQBP1 is responsible for the biological dysfunctions underlying mental retardation disorders [12] , [19] , [20] , [21] , [22] . In the present study, we determined the structure of the ternary complex of PQBP1-CT37, U5–15kD and the GYF domain of U5–52K, as well as the binary complex of PQBP1-CT43 and U5–15kD. Our data suggest that the ternary complex of PQBP1, U5–15kD and U5–52K is integrated into the spliceosome. The ternary complex would be disrupted by the loss of the YxxPxxVL motif, leading to destabilization of the spliceosome. In order to fully understand the mechanism by which the PQBP1 loss of function leads to mental retardation, it will be necessary to investigate how the deletion of the YxxPxxVL motif destabilizes the spliceosome and its effects on pre-mRNA splicing in cell culture and in vivo . There are seven frameshift mutations in the PQBP1 gene that have been identified in families with XLMR [10] , [11] , [12] , [13] , [15] , [16] , [17] , [18] . We demonstrate here that all the frameshift mutations reported so far cause the loss of the YxxPxxVL motif that is essential for the U5–15kD binding. This strongly suggests that the loss of the YxxPxxVL motif is responsible for XLMR induced by the PQBP1 frameshifts. In addition to the frameshift mutations, the R196Stop missense mutation, Y65C missense mutation, and two different deletions of seven amino acids (residues 112–118 or residues 132–138) have been associated with the XLMR disorders. It is important to note that the deletions of seven amino acids were found in controls, and thus these deletions may be non-pathogenic or could act subtly on PQBP1 function [10] . The R196Stop missense mutation causes the loss of the YxxPxxVL motif, which is essential for the interaction with U5–15kD [11] . However, the Y65C missense mutation occurs in the WW domain [14] , and the PQBP1-Y65C mutant completely retains the YxxPxxVL motif. Furthermore, the Y65C mutation blocks the ability of PQBP1 to interact with WBP11/NpwBP/SIPP1 and Dynamin 2 (refs 21 , 31 ). Therefore, the YxxPxxVL motif of PQBP1 is not the only functional element that is compromised in the pathogenesis of XLMR. From these findings, we conclude that PQBP1 requires the WW domain and the YxxPxxVL motif in order to function properly: dysfunction of either functional element results in the XLMR disorders. In the nucleus, the N-terminal WW domain binds to the splicing factor WBP11 (ref. 9 ), whereas the C-terminal YxxPxxVL motif binds to the spliceosomal protein U5–15kD [6] , [7] , [8] . PQBP1, WBP11 and U5–15kD are all components of the precatalytic B complex [4] , [5] , and thus PQBP1 probably binds to both WBP11 and U5–15kD in the B complex. Sudol et al. [32] suggested the possibility that PQBP1(236–247) interacts with the WW domain in an intra-molecular manner. This region includes the sequence GPLFQQRPYPSPG that contains a part of the YxxPxxVL motif. It might be expected, therefore, that PQBP1 would be auto-inhibited by the intra-molecular interaction between the N-terminal WW domain and the C-terminal region [32] . In order to examine the possibility of such auto-inhibition, we investigated the interaction between the WW domain and the YxxPxxVL motif using nuclear magnetic resonance (NMR) spectroscopy ( Supplementary Fig. 4 ). The solution NMR technique is sensitive for detecting weak interactions between proteins: it can detect the interactions with a K D value in the millimolar range [33] . However, no significant chemical shift change was observed in the presence of an excess amount of PQBP1-CT43 ( Supplementary Fig. 4 ). Furthermore, full-length PQBP1 binds to U5–15kD with a K D value similar to that of PQBP1-CT43. Therefore, it is unlikely that PQBP1 is auto-inhibited by an intra-molecular interaction, although we cannot rule out the possibility that the WW domain interacts very weakly with the C-terminal region. These observations are compatible with the small angle X-ray scattering study of PQBP1 reported by Ree et al. [34] PQBP1 has an elongated shape with a Stokes radius of 3.7 nm and a maximum molecular dimension of 13 nm [34] . Although PQBP1 is not conserved in yeast, U5–15kD is highly conserved from yeast to humans [8] . The U5–15kD ortholog from Saccharomyces cerevisiae , called Dib1p, is essential for pre-mRNA splicing in vivo [8] . Dib1p shares a sequence identity of 66% with human U5–15kD, and conserves the residues forming the hydrophobic groove of U5–15kD, which is the interface for the interaction with the YxxPxxVL motif [8] . PQBP1 is a component of the Prp19 complex, whereas U5–15kD and U5–52K are both U5 snRNP components [4] , [5] , [35] . Hoskins et al. [36] have shown that the PrP19 complex joins the spliceosome after the U4/U6.U5 tri-snRNP recruitment. This means that PQBP1 also joins the spliceosome after the tri-snRNP recruitment. Therefore, our results suggest that the YxxPxxVL motif in PQBP1 contributes to the association of the PrP19 complex with the U5 snRNP. As described in the Results section, the affinities of U5–15kD for PQBP1 and for U5–52K are weak. A weak binding affinity is important for dynamic spliceosome assembly, and is a common characteristic of pre-mRNA splicing factors [35] . Protein expression and purification We used U5–15kD(4–137) lacking the N-terminal three residues and the C-terminal five residues. The DNAs encoding U5–15kD(4–137), U5–15kD(4–137)-PQBP1(223–265) and U5–15kD(4–137)-PQBP1(229–265) were inserted into a pOPTH plasmid. The DNAs encoding full-length PQBP1 and the GYF domain of U5–52K (residues 280–341) were also inserted into a pOPTH plasmid. The DNA encoding PQBP1(223–265) was inserted into a pOPTG plasmid. The DNA encoding PQBP1(36–94) was inserted into a pGEX-2TK plasmid [23] . All constructs were verified by DNA sequencing. The proteins were expressed in C41(DE3)RIPL or BL21(DE3) cells harbouring the pOPTG, pOPTH or pGEX-2TK plasmid. Protein expression was induced by the addition of isopropyl-β-D-thiogalactopyranoside at a final concentration of 0.3 mM. After 3 h cultivation, the cells were collected by centrifugation at 3,765 g for 15 min at 4 °C. The full-length PQBP1, U5–15kD(4–137), U5–15kD(4–137)-PQBP1(223–265), U5–15kD(4–137)-PQBP1(229–265) and U5–52K(280–341) were expressed with an N-terminal His-tag (MAHHHHHHM). The C41(DE3)RIPL cells were resuspended in buffer A (20 mM Tris-HCl, 100 mM NaCl and 20 mM imidazole at pH 8.0) and lysed by sonication on ice. The proteins were detected in a soluble fraction after centrifugation at 9,400 g for 60 min at 4 °C. The His6-tagged proteins were purified with an Ni-NTA agarose column (Qiagen) equilibrated with buffer A, followed by further purification by gel filtration on a Superdex 75 16/60 column (GE Healthcare Bio Sciences) equilibrated with buffer B (20 mM Tris–HCl, 100 mM NaCl and 1 mM dithiothreitol at pH 8.5) or buffer C (10 mM Tris–HCl, 150 mM NaCl and 3 mM EDTA at pH 8.5). PQBP1-CT43 was expressed as a glutathione S-transferase (GST)-fusion protein. The C41(DE3)RIPL cells were resuspended in buffer D (20 mM Tris–HCl, 100 mM NaCl and 1 mM dithiothreitol at pH 7.5) and lysed by sonication on ice. The proteins were detected in a soluble fraction after centrifugation at 9,400 g for 60 min at 4 °C. The GST-fusion proteins were purified with a glutathione Sepharose 4B column (GE Healthcare Bio Sciences) equilibrated with buffer D. The purified GST-fusion protein was digested with TEV protease for 15 h at 4 °C to remove the GST region. Thereafter, the proteins were purified by high-performance liquid chromatography. The purified PQBP1-CT43 has an N-terminal extension (GSHM) derived from the pOPTG plasmid. PQBP1(36–94) was also expressed as a GST-fusion protein. The BL21(DE3) cells were grown in M9 minimal medium supplemented with 15 NH 4 Cl. Thrombin was used for cleavage of GST-PQBP1(36–94). PQBP1(36–94) was purified by gel-filtration chromatography [23] . Crystallization Before crystallization, the protein solution buffer was changed to buffer B by gel filtration or dialysis. Optimal crystals for the complex of PQBP1-CT43 with U5–15kD were obtained at 20 °C by the sitting drop vapour diffusion method from a protein solution at 8.1 mg ml −1 containing a 1:5 molar ratio of U5–15kD:PQBP1-CT43 and a reservoir solution containing 15% PEG3350 and 0.1 M sodium acetate at pH 6.5. Crystals were cryoprotected by adding glycerol to a final concentration of 20% and frozen in liquid nitrogen. The fusion protein of U5–15kD(4–137) and PQBP1-CT43 was crystallized at 20 °C by the sitting drop vapour diffusion method from a protein solution at 12.2 mg ml −1 and a reservoir solution containing 0.1 M sodium acetate at pH 4.2 and 0.5 M NaCl. Crystals were cryoprotected by adding glycerol to a final concentration of 30% and frozen in liquid nitrogen. The complex of U5–15kD-PQBP1-CT37 and the GYF domain of U5–52K was crystallized at 20 °C by the sitting drop vapour diffusion method from a protein solution at 11.9 mg ml −1 containing a 1:1 molar ratio of U5–15kD-PQBP1-CT37:GYF and a reservoir solution containing 0.7 M ammonium sulphate at pH 5.3. The crystals were cryoprotected by adding glycerol to a final concentration of 25% and frozen in liquid nitrogen. Crystallographic structure determination Diffraction data were collected at 100 K on Beamlines BL41XU and BL38B1 at Spring8 (Harima, Japan). Data processing and scaling were done with iMosflm and Scala. The crystallographic phase problem was solved by means of molecular replacement. The structures were manually rebuilt with Coot [37] and refined with Refmac [38] . The final models of the binary complex had 97.6% of residues in the core areas of the Ramachandran plot with no residues in disallowed regions. The final models of the fusion protein of U5–15kD(4–137) and PQBP1-CT43 had 97.3% of residues in the core areas of the Ramachandran plot with no residues in disallowed regions. The Ramachandran plot for the ternary complex had 90.8% of residues in the core regions and none in disallowed regions. The data collection and refinement statistics are given in Table 1 . Figures depicting the structure were prepared with the program PyMOL (Delano Scientific). Structural coordinates have been deposited in the Protein Data Bank (PDB accession numbers 4BWQ, 4BWS and 4CDO). SPR measurements U5–15kD(4–137) was engineered to have a His6-tag (MAHHHHHH) followed by a biotinylation-tag (SSGSLHHILDAQKMVWNHRHM) at the N terminus. The biotinylation-tag sequence allows biotinylation of a single lysine residue by biotin–protein ligase. The biotin–protein ligase BirA500 (Avidity) was used to biotinylate the His6-biotinylation-tagged protein in the presence of biotin and ATP according to the manufacturer's protocol. After biotinylation, the protein was purified by gel filtration on a Superdex 75 16/60 column equilibrated with buffer C. Approximately 1,200 resonance units of the biotinylated U5–15kD were immobilized on the CM5 chip, onto which streptavidin had been covalently coupled via amine coupling. Biotinylated bovine serum albumin was prepared with biotinamidohexanoic acid N -hydroxysuccinimide ester (Sigma-Aldrich). The biotinylated bovine serum albumin was immobilized in a reference flow cell to eliminate the effects of nonspecific binding [39] . A BIAcore J instrument (GE Healthcare) was used for SPR measurements, all of which were carried out at 25 °C with a constant flow rate of 30 μl min −1 . The solution contained 10 mM Tris–HCl (pH 8.5), 150 mM NaCl, 3 mM EDTA and 0.005% Tween 20. All SPR measurements were performed at pH 8.5, which prevents protein aggregation at high concentrations of PQBP1-CT43. PQBP1-CT43 or the GYF domain of U5–52K was injected over sensor surfaces on which biotinylated U5–15kD or biotinylated BSA had been immobilized. Because the binding was saturated 100 s after the injection, we performed equilibrium binding analysis to quantify the interactions [39] . The binding response at equilibrium was calculated by subtracting the equilibrium response measured in the reference flow cell from that in the U5–15kD-immobilized flow cell. The equilibrium dissociation constants ( K D ) were determined by the nonlinear least squares method assuming a 1:1 Langmuir binding model. The SPR measurements for the binding of the GYF domain to biotinylated U5–15kD-PQBP1-CT43 were performed in the same manner. Fluorescence measurements Full-length PQBP1 was titrated into 400 μl solution (20 mM Tris–HCl and 100 mM NaCl at pH 8.5) containing 159 nM U5–15kD(4–137), which was labelled with Lumio Green (FlAsH) at the N terminus. Fluorescence anisotropy was measured with an F-4500 fluorescence spectrophotometer (Hitachi) at 25 °C with an excitation wavelength of 490 nm and an emission wavelength of 530 nm. Excitation and emission slits were set at 10 nm. The K D values were determined by the nonlinear least squares method assuming a 1:1 binding model. Binding of PQBP1-CT43 to FlAsH-tagged U5–15kD did not change the fluorescence anisotropy, as PQBP1-CT43 is rather small. The total fluorescence intensity was used to determine the K D value between PQBP1-CT43 and FlAsH-tagged U5–15kD. NMR spectroscopy The NMR sample contained 30 μM 15 N-labelled PQBP1(36–94), 150 μM PQBP1-CT43, 10 mM sodium phosphate (pH 7.0), 1 mM dithiothreitol, 5% D 2 O, 1 mM NaN 3 and 20 μM 2,2-dimethyl-2-silapentane-5-sulphonate sodium salt. NMR experiments were performed at 288K on a Bruker Avance 800 MHz spectrometer equipped with a cryoprobe. Accession codes. Atomic coordinates and structure factors have been deposited in the Protein Data Bank under accession codes 4BWQ (binary complex), 4BWS (ternary complex) and 4CDO (the fusion protein of U5–15kD and PQBP1-CT43). How to cite this article: Mizuguchi, M. et al. Mutations in the PQBP1 gene prevent its interaction with the spliceosomal protein U5–15kD. Nat. Commun. 5:3822 doi: 10.1038/ncomms4822 (2014).